A RIPK2 inhibitor delays NOD signalling events yet prevents inflammatory cytokine production Intracellular nucleotide binding and oligomerization domain (NOD) receptors recognize antigens including bacterial peptidoglycans and initiate immune responses by triggering the production of pro-inflammatory cytokines through activating NF-κB and MAP kinases. Receptor interacting protein kinase 2 (RIPK2) is critical for NOD-mediated NF-κB activation and cytokine production. Here we develop and characterize a selective RIPK2 kinase inhibitor, WEHI-345, which delays RIPK2 ubiquitylation and NF-κB activation downstream of NOD engagement. Despite only delaying NF-κB activation on NOD stimulation, WEHI-345 prevents cytokine production in vitro and in vivo and ameliorates experimental autoimmune encephalomyelitis in mice. Our study highlights the importance of the kinase activity of RIPK2 for proper immune responses and demonstrates the therapeutic potential of inhibiting RIPK2 in NOD-driven inflammatory diseases. NOD1 and NOD2 are cytosolic receptors of the innate immune system, able to sense bacterial peptidoglycans from Gram positive and Gram negative bacteria [1] , [2] , [3] . Their function in innate immune responses has been extensively studied, revealing pivotal roles in host defense against pathogens such as Listeria monocytogenes , Helicobacter pylori and Staphylococcus aureus [4] , [5] , [6] . In humans, deregulated NOD signalling due to mutations in NOD receptors, particularly in NOD2, are associated with Crohn’s disease, an inflammatory gastrointestinal disorder [7] , [8] , [9] . Aberrant activation of the NOD pathway can result in Blau syndrome or early-onset sarcoidosis, both characterized by familial granulomatous arthritis and skin granulomas [10] . Recently, a crucial role for receptor interacting kinase 2 (RIPK2) in promoting infiltration of immune cells into the central nervous system (CNS) was reported and RIPK2-deficient mice displayed reduced disease development and progression in a murine model for multiple sclerosis [11] . Once activated, NOD signalling leads to the activation of NF-κB and MAP kinases resulting in the transcription of pro-inflammatory cytokines [12] , as well as the induction of autophagy [13] . Multiple components and regulators of the NOD signalling complex have recently been described. RIPK2 plays a central role in the NOD signalling pathway and cells deficient in RIPK2 fail to mount a cytokine response upon NOD stimulation [14] , [15] . We and others have shown that upon NOD stimulation, RIPK2 is ubiquitylated by inhibitor of apoptosis (IAP) proteins, and this recruits the linear ubiquitination assembly complex (LUBAC), which is essential for downstream signalling [16] , [17] , [18] . While the role of RIPK2 as a NOD adaptor protein and ubiquitylation platform has been established, the biological role and function of RIPK2 as a kinase remains enigmatic. RIPK2 was originally identified as a serine–threonine kinase based on sequence homology [19] , [20] , [21] , but has recently been reclassified as a dual-specificity kinase [22] . Earlier reports suggested that the kinase activity of RIPK2 was dispensable for NF-κB activation and cytokine production [23] . On the other hand, a kinase-dead (K47A) knock-in mouse was developed and bone marrow-derived macrophages (BMDMs) derived from this mouse were defective in signalling [24] ; however, mutant RIPK2 was not expressed at detectable levels suggesting that kinase activity is required for stable expression rather than signalling per se [24] . Upon activation, RIPK2 autophosphorylates on Ser176 and on Tyr474 (refs 22 , 25 ). While Ser176 phosphorylation is essential for RIPK2 activity, phosphorylation of Tyr474 enhances, but is not essential for signalling [22] . Several kinase inhibitors have been described to inhibit RIPK2, albeit non-selectively. Among them are the epidermal growth factor receptor (EGFR) tyrosine kinase inhibitors Gefitinib and Eroltinib [22] and the p38, mitogen-activated protein kinase (MAPK) and Src inhibitor SB-203580 (refs 26 , 27 ). Pharmacological inhibition of RIPK2 kinase activity via these relatively nonspecific inhibitors caused a reduction in RIPK2 stability and a reduction in cytokine production upon NOD stimulation. However, these inhibitors also inhibit other kinases in the NOD signalling pathway to varying degrees; therefore, it is difficult to distinguish RIPK2-specific effects. To better understand the role of the kinase activity of RIPK2 in NOD signalling and to explore RIPK2 as a potential therapeutic target, we developed a specific and potent RIPK2 inhibitor and tested it in vitro and in vivo . WEHI-345 is a potent and selective inhibitor of RIPK2 A potent and specific RIPK2 inhibitor was identified by screening a proprietary library of 120 kinase inhibitors. This compound, WEHI-345 ( Fig. 1a ), is an ATP analogue and was therefore predicted to bind in the ATP-binding pocket of RIPK2. 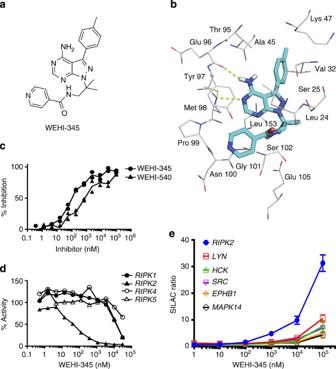Figure 1: WEHI-345 is a selective inhibitor of RIPK2. (a) Chemical structure of WEHI-345. (b) Model of WEHI-345 docked into the putative ATP-binding pocket of RIPK2. Displayed are the amino acids (shown as a line representation), which interact with WEHI-345 (shown as stick representation). Colour coding: carbon in grey for RIP2 and cyan for WEHI-345, hydrogen in grey, oxygen in red, nitrogen in blue and sulfur in yellow. Hydrogen bonds are highlighted as yellow dashed lines. (c)In vitrokinase assay using recombinant RIPK2. Values were normalized to RIPK2 activity in the absence of inhibitor. IC50(WEHI-345)=0.13 μM, IC50(WEHI-540)=1.01 μM. Technical duplicates of one out of three assays are shown. (d) Inhibition of RIP kinases by WEHI-345 determined by in vitrokinase assay using recombinant RIPK1, -2, -4 and -5. (e) SILAC-labelled THP-1 cells were lysed and treated with increasing concentrations of WEHI-345 before precipitation with Sepharose bound WEHI-345. SILAC ratios of the six strongest binders are shown as average and range of two technical repeats. Average SILAC ratios and ranges of all identified proteins are available asSupplementary Data set. Figure 1: WEHI-345 is a selective inhibitor of RIPK2. ( a ) Chemical structure of WEHI-345. ( b ) Model of WEHI-345 docked into the putative ATP-binding pocket of RIPK2. Displayed are the amino acids (shown as a line representation), which interact with WEHI-345 (shown as stick representation). Colour coding: carbon in grey for RIP2 and cyan for WEHI-345, hydrogen in grey, oxygen in red, nitrogen in blue and sulfur in yellow. Hydrogen bonds are highlighted as yellow dashed lines. ( c ) In vitro kinase assay using recombinant RIPK2. Values were normalized to RIPK2 activity in the absence of inhibitor. IC 50 (WEHI-345)=0.13 μM, IC 50 (WEHI-540)=1.01 μM. Technical duplicates of one out of three assays are shown. ( d ) Inhibition of RIP kinases by WEHI-345 determined by i n vitro kinase assay using recombinant RIPK1, -2, -4 and -5. ( e ) SILAC-labelled THP-1 cells were lysed and treated with increasing concentrations of WEHI-345 before precipitation with Sepharose bound WEHI-345. SILAC ratios of the six strongest binders are shown as average and range of two technical repeats. Average SILAC ratios and ranges of all identified proteins are available as Supplementary Data set . Full size image To gain insights into how WEHI-345 engages the RIPK2 kinase domain, we generated a structural model of the murine RIPK2 kinase domain (residues 18–249), the focus of the present work, using the unpublished X-ray crystal structure of human RIPK2 in complex with ponatinib (PDB: 4C8B) and the Necrostatin-1 bound murine RIPK1 structure (PDB ID: 4ITH [28] ) as templates. As is common among inactive protein kinases structures, the hRIPK2 activation loop (residues 165–188) was largely absent, so modelling utilized the structure of murine RIPK1, where only 13 amino acids were absent in this region. The stereochemical quality of the resultant model was assessed via Procheck [29] , which showed that over 97% of the amino acids resided in the allowed regions of the Ramachandran plot. Computational docking of WEHI-345 into this murine RIPK2 homology model is consistent with WEHI-345 occupation of the ATP-binding pocket of RIPK2 with hydrogen bonds between the adenosine ring of WEHI-345 and the hinge region residues Glu96 and Met98 of RIPK2 ( Fig. 1b ). The docking predicts that the adenosine ring of WEHI-345 is sandwiched between two leucine residues of RIPK2 (Leu24 and Leu153). There are numerous hydrophobic interactions between the inhibitor and RIPK2 involving residues; Leu24, Ser25, Val32, Ala45, Lys47, Thr95, Tyr97, Met98, Pro99, Asn100, Gly101, Ser102, Glu105 and Leu153, all contributing to the binding affinity between WEHI-345 and RIPK2. To have a less active control in our experiments, we designed a structurally related compound, WEHI-540 ( Supplementary Fig. 1a ). This compound contained a dimethyl amino group, which was predicted via computational docking to have less hydrophobic interactions with RIPK2 than the pyridine of WEHI-345 ( Supplementary Fig. 1b ). In a kinase assay, WEHI-345 inhibited the kinase activity of RIPK2 with an IC 50 of 130 nM ( Fig. 1c ), while WEHI-540 was approximately eightfold weaker in inhibiting RIPK2 (IC 50 =1.01 μM). The family of RIP kinases is characterized by their relatively conserved kinase domain [30] , [31] , [32] . We therefore tested the activity of WEHI-345 against other RIPKs in a KINOMEscan. WEHI-345 proved to be highly specific for RIPK2 ( K d =46 nM) and displayed negligible activity (>10 μM) against RIPK1, RIPK4 and RIPK5 ( Fig. 1d ). To confirm the absence of activity towards RIPK1, which is also associated with the NODosome [17] and plays an important role in other innate immune signalling pathways, we performed an in vitro kinase assay with immunoprecipitated RIPK1 from immortalized mouse BMDMs. Addition of ATP to RIPK1 promoted rapid auto-Ser/Thr phosphorylation and this autophosphorylation was blocked by the RIPK1 inhibitor Nec-1. Neither WEHI-345 nor WEHI-540 at a concentration of 1 μM was able to prevent autophosphorylation of RIPK1 ( Supplementary Fig. 1c ), indicating a lack of activity towards this kinase. RIPK3 activity was assessed using mouse dermal fibroblasts (MDFs), treated with a cocktail of tumour necrosis factor (TNF), Smac-mimetic compound A (cA) and the pan-caspase inhibitor Q-VD-OPh. This treatment induces necroptosis that is dependent on the kinase activities of RIPK1 and RIPK3 and the pseudokinase mixed lineage kinase domain-like (MLKL) [33] , [34] , [35] . While the RIPK1 inhibitor Necrostatin-1 significantly reduced necroptosis, neither WEHI-345 nor WEHI-540 had any effect on cell death, ruling out activity of WEHI-345 against RIPK1, RIPK3 or MLKL ( Supplementary Fig. 1d ) at 500 nM. To obtain a complete picture of the inhibitory profile of WEHI-345 in cells, we prepared a derivative of WEHI-345 that was linked via an amino group to sepharose beads and used it to precipitate and identify intracellular targets of our drug. Lysates of SILAC-labelled THP-1 cells were pretreated with increasing amounts of unbound WEHI-345 and binding partners in either pretreated or untreated lysates were precipitated with sepharose bound WEHI-345. Differentially labelled untreated and precompeted precipitates were then mixed and subjected to analysis by mass spectrometry [36] . Precompetition with WEHI-345 led to a large increase in the SILAC ratio for RIPK2. Smaller increases were also observed for LYN, HCK, SRC, EPHB1 and MAPK14 (p38) in that order ( Fig. 1e , Supplementary Data set 1 ). Notably, at a concentration of 1 μM of free drug, the only identified target of WEHI-345 was RIPK2. We also tested 92 kinases using KINOMEscan ( Supplementary Table 1 ). At a concentration of 1 μM, WEHI-345 showed activity of higher than 90% inhibition towards only four tested recombinant kinases (KIT, RET, PDGFRß and SRC) and an inhibition of more than 65% for a total of six tested kinases (S(35)=0.067). It is worth noting that the sixth strongest hit in the SILAC experiment (MAPK14, p38) was only detected at 100 μM of free drug and was not inhibited at all in the KINOMEscan. Together these data show that WEHI-345 is a highly specific inhibitor for RIPK2 and that in the monocyte cell lines used for NOD assays that RIPK2 is its only real target. Compared with the widely used RIPK2 inhibitors SB-203580 and Erlotinib, WEHI-345 has negligible activity against p38 and epidermal growth factor receptor (EGFR). Inhibition of Src by WEHI-345 is, however, similar to SB-203580 ( Supplementary Table 1 ). Thus, WEHI-345 has a superior and unique kinase inhibition profile than previously described inhibitors of RIPK2 in terms of specificity and selectivity. WEHI-345 is non-cytotoxic and active in cultured cells Neither WEHI-345 nor WEHI-540 was cytotoxic to BMDMs when used at concentrations of up to 1 μM in combination with NOD stimulation ( Fig. 2a ). To confirm the activity of WEHI-345 in a cellular context, we immunoprecipitated phospho-RIPK2 using an RIPK2 P-Ser176-specific antibody from unstimulated and MDP-stimulated cells ( Fig. 2b ). We were able to immunoprecipitate small amounts of autophosphorylated RIPK2 from unstimulated BMDMs; however, addition of MDP markedly increased the amounts of Ser176 phosphorylated RIPK2. Pretreatment with WEHI-345 reduced the levels of P-Ser176-RIPK2 to levels seen in unstimulated cells demonstrating that WEHI-345 is able to inhibit MDP-induced autophosphorylation activity of RIPK2 in cells. 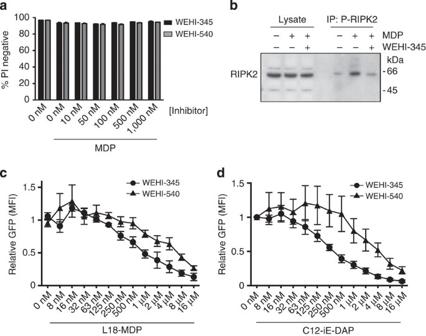Figure 2: WEHI-345 is not cytotoxic and inhibits RIPK2 activity in cells. (a) Cell survival was assessed on MDP and WEHI-345, respectively WEHI-540 stimulated BMDMs using PI staining and flow cytometry 24 h after treatment.n=3. (b) Raw 267.4 cells were either left untreated, treated with 10 μg ml−1MDP or with 500 nM WEHI-345 and MDP. Lysates were immunoprecipitated using a P-Ser176-specific RIPK2 antibody. Levels of RIPK2 in lysates and immunoprecipitations were determined using western blot for total RIPK2. One representative experiment of three repeats is shown. (c,d)In vitroactivity of WEHI-345 and WEHI-540 in L18-MDP (200 ng ml−1) (c) or C12 DAP (1 μg ml−1) (d) stimulated THP-1 cells was tested using a NF-κB-GFP reporter assay. Values were normalized to untreated (0%) and L18-MDP, respectively, C12-iE-DAP-treated cells (100%).n≥3. Error bars are s.e.m. Figure 2: WEHI-345 is not cytotoxic and inhibits RIPK2 activity in cells. ( a ) Cell survival was assessed on MDP and WEHI-345, respectively WEHI-540 stimulated BMDMs using PI staining and flow cytometry 24 h after treatment. n =3. ( b ) Raw 267.4 cells were either left untreated, treated with 10 μg ml −1 MDP or with 500 nM WEHI-345 and MDP. Lysates were immunoprecipitated using a P-Ser176-specific RIPK2 antibody. Levels of RIPK2 in lysates and immunoprecipitations were determined using western blot for total RIPK2. One representative experiment of three repeats is shown. ( c , d ) In vitro activity of WEHI-345 and WEHI-540 in L18-MDP (200 ng ml −1 ) ( c ) or C12 DAP (1 μg ml −1 ) ( d ) stimulated THP-1 cells was tested using a NF-κB-GFP reporter assay. Values were normalized to untreated (0%) and L18-MDP, respectively, C12-iE-DAP-treated cells (100%). n ≥3. Error bars are s.e.m. Full size image We then assessed the role of the kinase activity of RIPK2 in NOD signalling using WEHI-345. THP-1 cells were stably infected with a lentiviral NF-κB green fluorescent protein (GFP) reporter and pretreated with WEHI-345 or WEHI-540 before stimulation with either L18-MDP ( Fig. 2c ) or C12-iE-DAP ( Fig. 2d ). WEHI-345 reduced reporter activity compared with untreated cells at concentrations above 100 nM. As expected, WEHI-345 was more potent than WEHI-540 in inhibiting NOD1- and NOD2-dependent NF-κB activity. WEHI-345 inhibits cytokine production upon NOD stimulation WEHI-345 potently blocked MDP-induced transcription of the inflammatory mediators TNF and interleukin-6 (IL-6) in BMDMs ( Fig. 3a,b ). Similarly, in WEHI-345-treated THP-1 cells stimulated with MDP we observed reduced mRNA levels of NF-κB targets such as TNF, IL-8, IL-1β and A20 ( Fig. 3c,d ; Supplementary Fig. 2a,b ) demonstrating that WEHI-345 inhibits both human and mouse RIPK2-dependent inflammatory cytokine transcription. 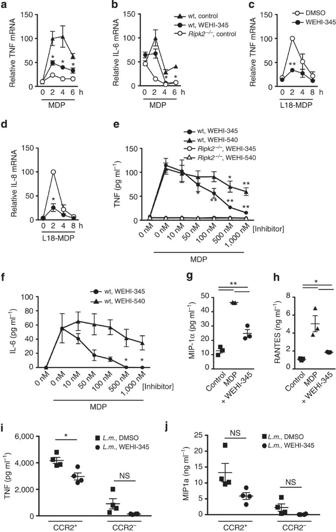Figure 3: WEHI-345 blocks cytokine transcription and secretion on NOD stimulation and bacterial infection. (a,b) Interferonγ (IFNγ)-primed BMDMs from wild-type orRipk2−/−mice were stimulated with 10 μg ml−1MDP in the absence or presence of WEHI-345 (500 nM) and RNA levels of TNF (a) and IL-6 (b) were determined using reverse transcription (RT)–qPCR.n=3. (c,d) THP-1 cells were stimulated with 200 ng ml−1L18-MDP in the presence or absence of WEHI-345 (2 μM) and mRNA levels of TNF (c) and IL-8 (d) were determined using RT–PCR,n=3, target accumulation at 2 h in L18-MDP+vehicle-treated cells was set to 100%. (e,f) IFNγ-primed wild-type BMDMs (n=6) were treated with increasing concentrations of WEHI-345 for 30 min before the addition of MDP and levels of TNF (e), and IL-6 (f), were measured using enzyme-linked immunosorbent assay 24 h after the addition of MDP. RIPK2−/−BMDMs (n=1) were used as a negative control. (g,h) MIP-1α (g) and RANTES (h) levels in the supernatant of IFNγ-primed BMDMs were measured from untreated, MDP (10 μg ml−1) stimulated or WEHI-345 (500 nM)+MDP-treated BMDMs of wild-type mice.n=3. (i,j) CCR2+and CCR2−monocytes were infected withListeria monocytogenesand cytokine levels in the supernatant were measured using Bioplex analysis.n=4. In all panels, * indicatePvalues <0.05 and ** indicatePvalues <0.005 based on a non-paired Student’st-test for control versus drug treated samples of one time point or one concentration. Error bars are s.e.m. Figure 3: WEHI-345 blocks cytokine transcription and secretion on NOD stimulation and bacterial infection. ( a , b ) Interferonγ (IFNγ)-primed BMDMs from wild-type or Ripk2 −/− mice were stimulated with 10 μg ml −1 MDP in the absence or presence of WEHI-345 (500 nM) and RNA levels of TNF ( a ) and IL-6 ( b ) were determined using reverse transcription (RT)–qPCR. n =3. ( c , d ) THP-1 cells were stimulated with 200 ng ml −1 L18-MDP in the presence or absence of WEHI-345 (2 μM) and mRNA levels of TNF ( c ) and IL-8 ( d ) were determined using RT–PCR, n =3, target accumulation at 2 h in L18-MDP+vehicle-treated cells was set to 100%. ( e , f ) IFNγ-primed wild-type BMDMs ( n =6) were treated with increasing concentrations of WEHI-345 for 30 min before the addition of MDP and levels of TNF ( e ), and IL-6 ( f ), were measured using enzyme-linked immunosorbent assay 24 h after the addition of MDP. RIPK2 −/− BMDMs ( n =1) were used as a negative control. ( g , h ) MIP-1α ( g ) and RANTES ( h ) levels in the supernatant of IFNγ-primed BMDMs were measured from untreated, MDP (10 μg ml −1 ) stimulated or WEHI-345 (500 nM)+MDP-treated BMDMs of wild-type mice. n =3. ( i , j ) CCR2 + and CCR2 − monocytes were infected with Listeria monocytogenes and cytokine levels in the supernatant were measured using Bioplex analysis. n =4. In all panels, * indicate P values <0.05 and ** indicate P values <0.005 based on a non-paired Student’s t -test for control versus drug treated samples of one time point or one concentration. Error bars are s.e.m. Full size image MDP-induced secretion of the pro-inflammatory cytokines TNF and IL-6 ( Fig. 3e,f ) and chemokines MIP-1α, RANTES ( Fig. 3g,h ) and monocyte chemoattractant protein-1 (MCP-1; Supplementary Fig. 2c ) was also potently inhibited at submicromolar concentrations of WEHI-345 in interferon-γ-primed BMDMs. Consistent with our biochemical analysis, WEHI-540 was 10-fold weaker in reducing secretion of cytokines in BMDMs. Ripk2 −/− BMDMs did not induce any cytokines or chemokines confirming the RIPK2-dependent nature of our NOD stimulation protocol. WEHI-345 also potently inhibited MDP-induced cytokine and chemokine secretion in the mouse macrophage Raw 264.7 cell line ( Supplementary Fig. 2d,e ). To test the efficacy of WEHI-345 to inhibit pathogen-induced activation of NOD pathways, we infected CD11β + monocytes with Listeria monocytogenes and measured cytokine secretion in both CCR2 − and CCR2 + subsets, as this stimulus has been reported to induce RIPK2-dependent cytokine production [5] . In both subsets, Listeria infection induced a cytokine (represented by TNF) and chemokine (represented by MIP-1α) response when compared with untreated controls. CCR2 − and CCR2 + monocytes from RIPK2-deficient animals secreted less cytokines and chemokines on Listeria infection compared with wild-type cells ( Supplementary Fig. 2f,g ) confirming that Listeria activates NOD signalling pathways. Consistent with a role for RIPK2 in response to an infection, we observed a trend towards reduced cytokine and chemokine secretion upon WEHI-345 pretreatment ( Fig. 3i,j ), that was statistically significant in the case of Listeria -induced TNF secretion from the CCR2 + monocyte population. As a wide variety of stimuli induce a cytokine response in macrophages and monocytes, we tested the ability of WEHI-345 to prevent cytokine production by BMDMs induced by other inflammatory stimuli. BMDMs were treated with MDP, TNF, smac-mimetic or lipopolysaccharide (LPS); all stimuli that result in cytokine secretion in this cell type, and levels of TNF and IL-6 were measured 24 h after stimulation ( Fig. 4a,b ). To enable comparison between stimuli despite their different potency to induce cytokines, we normalized values without inhibitor to 100% secretion for each stimulus. Addition of WEHI-345 significantly reduced the levels of TNF and IL-6 on MDP stimulation but had no effect on TNF, smac-mimetic or LPS stimulation. We observed a slight decrease of IL-6 levels upon the addition of WEHI-540 after LPS stimulation; however, this is unlikely to be due to RIPK2 inhibition. Neither WEHI-345 nor WEHI-540 had any effect on IL-1β production after treatment with the inflammasome stimuli Alum, ATP, smac-mimetic and Staurosporine ( Fig. 4c ). 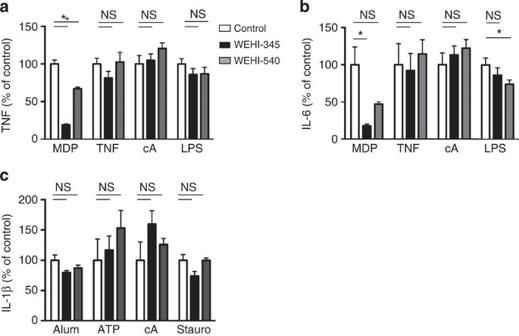Figure 4: WEHI-345 specifically blocks cytokine production on NOD stimulation. (a,b) Wild-type BMDMs were treated with IFNγ+MDP (10 μg ml−1), TNF (100 ng ml−1), Smac-mimetic (compound A, 500 nM) or LPS (2.5 ng ml−1). Cytokine levels of TNF (a,n=6–9) and IL-6 (b,n=3–6) were determined after 24 h by enzyme-linked immunosorbent assay (ELISA). Values were normalized to the average of control samples for better comparison. Absolute values of control samples for TNF (a) were: MDP: 142 pg ml−1, TNF: 29 pg ml−1, cA: 446 pg ml−1, LPS: 3.9 ng ml−1) and for IL-6 (b): MDP: 29 pg ml−1, TNF: 61 pg ml−1, cA: 188 pg ml−1, LPS: 12.9 ng ml−1). (c) Inflammasomes in LPS-primed wild-type BMDMs were activated using Alum (250 μg ml−1), ATP (5 mM), Smac-mimetic (Compound A, 500 nM) or Staurosporine (1 μM), and levels of IL-1β in the supernatant was measured by ELISA. Values were normalized to the average of control samples (Alum: 508 pg ml−1, ATP: 220 pg ml−1, compound A: 230 pg ml−1, Staurosporine: 124 pg ml−1).n=3–4. In all panels, * indicatePvalues <0.05 and ** indicatePvalues <0.005 based on a non-paired Student’st-test. Error bars are s.e.m. Figure 4: WEHI-345 specifically blocks cytokine production on NOD stimulation. ( a , b ) Wild-type BMDMs were treated with IFNγ+MDP (10 μg ml −1 ), TNF (100 ng ml −1 ), Smac-mimetic (compound A, 500 nM) or LPS (2.5 ng ml −1 ). Cytokine levels of TNF ( a , n =6–9) and IL-6 ( b , n =3–6) were determined after 24 h by enzyme-linked immunosorbent assay (ELISA). Values were normalized to the average of control samples for better comparison. Absolute values of control samples for TNF ( a ) were: MDP: 142 pg ml −1 , TNF: 29 pg ml −1 , cA: 446 pg ml −1 , LPS: 3.9 ng ml −1 ) and for IL-6 ( b ): MDP: 29 pg ml −1 , TNF: 61 pg ml −1 , cA: 188 pg ml −1 , LPS: 12.9 ng ml −1 ). ( c ) Inflammasomes in LPS-primed wild-type BMDMs were activated using Alum (250 μg ml −1 ), ATP (5 mM), Smac-mimetic (Compound A, 500 nM) or Staurosporine (1 μM), and levels of IL-1β in the supernatant was measured by ELISA. Values were normalized to the average of control samples (Alum: 508 pg ml −1 , ATP: 220 pg ml −1 , compound A: 230 pg ml −1 , Staurosporine: 124 pg ml −1 ). n =3–4. In all panels, * indicate P values <0.05 and ** indicate P values <0.005 based on a non-paired Student’s t -test. Error bars are s.e.m. Full size image In summary, our results demonstrate that WEHI-345 potently and specifically inhibits RIPK2 in cells to prevent NOD-induced cytokine production following MDP stimulation or bacterial infection. WEHI-345 delays NF-κB activation and RIPK2 ubiquitylation NOD-induced NF-κB reporter activity, cytokine mRNA levels and cytokine secretion was almost completely blocked by inhibition of the kinase activity of RIPK2 by WEHI-345. We therefore hypothesized that molecular markers of NF-κB activation would be absent in BMDMs treated with MDP and WEHI-345. To test this, we stimulated BMDMs with MDP and generated lysates at several time points post stimulation ( Fig. 5a ). Western blots of lysates from MDP-stimulated cells revealed a strong and reproducible phosphorylation of p65, IκBα and p38 after 30 min. Total IκBα levels were reduced at 60 min and returned to normal after 120 min, as expected. Intriguingly, given its ability to almost completely block cytokine production, WEHI-345 only delayed rather than blocked MDP-induced p65, IκBα and p38 phosphorylation and IκBα degradation. As expected, SB-203580, a low nanomolar K d inhibitor of p38, prevented MDP-induced phosphorylation of the p38 target MK-2. SB-203580 has also been reported to inhibit RIPK2 and interestingly, had a similar effect to WEHI-345 on the kinetics of IκBα degradation or p65, IκBα and p38 phosphorylation in response to MDP stimulation. To explore these unexpected observations, we performed the same experiment in the THP-1 cell line. As before, we observed a delay rather than a block of molecular markers for NF-κB and MAPK activation following WEHI-345 inhibition, although the inhibitor did reduce phosphorylation of JNK ( Fig. 5b ). This effect on delayed signalling observed with WEHI-345 was restricted to NOD stimulation and was not observed when cells were stimulated with LPS or TNF, even when a higher concentration of WEHI-345 was used ( Fig. 5c ). 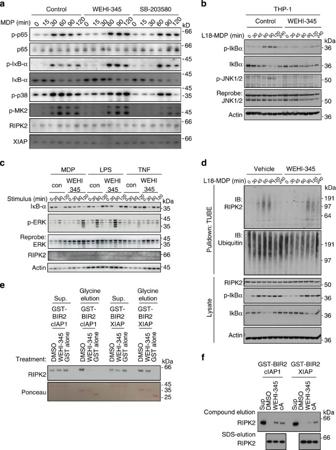Figure 5: Inhibition of RIPK2 activity delays NF-κB signalling and RIPK2 ubiquitination by interfering with IAP–RIPK2 interaction. (a) Interferonγ (IFNγ) primed wild-type BMDMs were either left untreated, treated with 500 nM WEHI-345 or SB-203580 30 min before the addition of 10 μg ml−1MDP. Cell lysates were taken at indicated time points after the addition of MDP and probed with the indicated antibodies. Probing for RIPK2 confirmed the genotype and β-actin blot was used as a loading control. One experiment out of six biologically independent cultures of BMDMs is shown. (b) THP-1 cells were either treated with WEHI-345 (2 μM) or left untreated 30 min before the addition of L18-MDP (200 nM). Cell lysates were taken at the indicated time points and probed for Phospho-IκBα, total-IκBα, Phospho-JNK1/2 and total JNK1/2 as a measure for NF-κB and MAPK activation. Actin was used as a loading control. One experiment out of three independent repeats is shown. (c) Wild-type BMDMs were either left untreated, treated with 1 μM WEHI-345 or WEHI-540 30 min before stimulation with IFNγ+MDP, LPS or TNF. Cell lysates from indicated time points were probed for NF-κB and MAPK activation with the indicated antibodies. One experiment out of six biologically independent cultures of BMDMs is shown. (d) THP-1 cells, either left untreated or pretreated with WEHI-345, were stimulated with L18-MDP for the indicated time points and ubiquitin conjugates were purified using TUBEs. Lysates and pull downs were tested by western blot using the indicated antibodies. One experiment out of two independent repeats is shown. (e) THP-1 cells were either left untreated or treated with WEHI-345 for 30 min before lysis. RIPK2 was precipitated using sepharose bound GST-BIR2 of cIAP1 or XIAP or GST alone and levels of precipitated RIPK2 was determined by western blot. Ponceau staining serves as a loading control for protein loading and GST conjugates. (f) RIPK2 was precipitated from THP-1 cells with sepharose bound GST-BIR2 of cIAP1 or XIAP and eluted using DMSO, WEHI-345 or the SMAC-mimetic, compound A (upper panel), followed by SDS elution (lower panel). Figure 5: Inhibition of RIPK2 activity delays NF-κB signalling and RIPK2 ubiquitination by interfering with IAP–RIPK2 interaction. ( a ) Interferonγ (IFNγ) primed wild-type BMDMs were either left untreated, treated with 500 nM WEHI-345 or SB-203580 30 min before the addition of 10 μg ml −1 MDP. Cell lysates were taken at indicated time points after the addition of MDP and probed with the indicated antibodies. Probing for RIPK2 confirmed the genotype and β-actin blot was used as a loading control. One experiment out of six biologically independent cultures of BMDMs is shown. ( b ) THP-1 cells were either treated with WEHI-345 (2 μM) or left untreated 30 min before the addition of L18-MDP (200 nM). Cell lysates were taken at the indicated time points and probed for Phospho-IκBα, total-IκBα, Phospho-JNK1/2 and total JNK1/2 as a measure for NF-κB and MAPK activation. Actin was used as a loading control. One experiment out of three independent repeats is shown. ( c ) Wild-type BMDMs were either left untreated, treated with 1 μM WEHI-345 or WEHI-540 30 min before stimulation with IFNγ+MDP, LPS or TNF. Cell lysates from indicated time points were probed for NF-κB and MAPK activation with the indicated antibodies. One experiment out of six biologically independent cultures of BMDMs is shown. ( d ) THP-1 cells, either left untreated or pretreated with WEHI-345, were stimulated with L18-MDP for the indicated time points and ubiquitin conjugates were purified using TUBEs. Lysates and pull downs were tested by western blot using the indicated antibodies. One experiment out of two independent repeats is shown. ( e ) THP-1 cells were either left untreated or treated with WEHI-345 for 30 min before lysis. RIPK2 was precipitated using sepharose bound GST-BIR2 of cIAP1 or XIAP or GST alone and levels of precipitated RIPK2 was determined by western blot. Ponceau staining serves as a loading control for protein loading and GST conjugates. ( f ) RIPK2 was precipitated from THP-1 cells with sepharose bound GST-BIR2 of cIAP1 or XIAP and eluted using DMSO, WEHI-345 or the SMAC-mimetic, compound A (upper panel), followed by SDS elution (lower panel). Full size image We and others have previously shown that RIPK2 is potently ubiquitylated on NOD stimulation, a process that is essential for the recruitment of linear ubiquitination assembly complex (LUBAC) to the signalling complex and efficient downstream signalling [17] , [37] . We therefore wanted to examine the role of RIPK2 kinase activity for its own ubiquitylation. Blocking RIPK2 kinase activity with WEHI-345 delayed RIPK2 ubiquitylation, which is consistent with the delay in activation of NF-κB in these cells ( Fig. 5d ). This links the activation of the NF-κB pathway very closely to the ubiquitylation of RIPK2 and suggests a tight crosstalk between kinase activity of RIPK2 and its own ubiquitylation. IAPs have been shown to be E3 ligases for RIPK2 and to interact via their BIR2 domain with the kinase domain of RIPK2 (refs 37 , 38 ). We therefore tested the hypothesis that WEHI-345 interferes with this interaction. Consistent with these earlier reports, sepharose-bound GST did not pull down RIPK2 from THP-1 cells, whereas glutathione sepharose bound GST-BIR2 from either cIAP1 or XIAP pulled down readily detectable amounts of RIPK2 ( Fig. 5e ). However, when cells were pretreated with WEHI-345 before lysis, the amount of RIPK2 that was pulled down by GST-BIR2 of cIAP1 was markedly reduced, indicating that WEHI-345 interferes with cIAP1–RIPK2 interaction ( Fig. 5e ). WEHI-345 was less potent in inhibiting the interaction between RIPK2 and the BIR2 of XIAP. To test this observation in another manner, we precipitated RIPK2 using GST-BIR2 of cIAP1 and XIAP from untreated THP-1 cells and eluted with either WEHI-345 or the SMAC-mimetic compound A, which binds to the BIR2 domains of IAPs [39] . Compared with compound A, WEHI-345 eluted equal amounts of RIPK2 from GST-BIR2 of cIAP1 and slightly lower amounts from GST-BIR2 of XIAP. These results suggest that WEHI-345 prevents the binding of IAPs to RIPK2, which could explain the delay in RIPK2 ubiquitylation and downstream signalling that we observed. WEHI-345 desynchronises transcriptional response Cytokine transcription, translation and secretion was almost completely blocked by WEHI-345; however, phosphorylation events within the NF-κB and p38 pathways were only delayed. We therefore tested whether the translocation to the nucleus of individual subunits of the NF-κB and activator protein-1 (AP-1) transcription factors was perturbed by WEHI-345 treatment and whether a desynchronization of these transcription factors could explain the loss of cytokine production in WEHI-345-treated cells. THP-1 cells were pretreated with WEHI-345 for 30 min followed by stimulation with L18-MDP for various time points. Cytoplasmic and nuclear extracts were prepared and examined for the NF-κB subunits p65, p50 and RelB as well as the AP-1 subunits cJun, cFos and JunB. All these transcription factor subunits were translocated to the nucleus after L18-MDP stimulation ( Fig. 6a ). Consistent with its effects on downstream signalling, WEHI-345 treatment delayed MDP-induced nuclear translocation of the NF-κB subunits p65 and p50 and JunB, but there was little evidence for such a delay for the AP-1 subunits cJun and cFos. 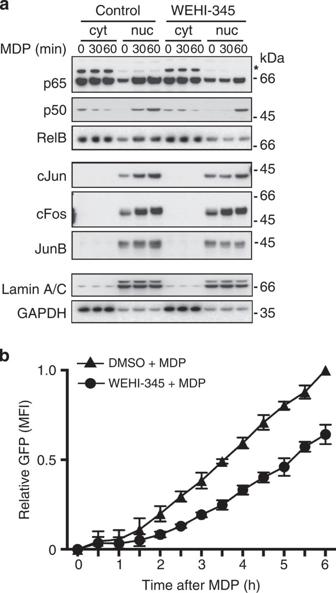Figure 6: WEHI-345 desynchronizes NF-κB and AP-1 transcription factors. (a) THP-1 cells were stimulated with 200 ng ml−1L18-MDP for the indicated time points, cytoplasmic and nuclear fractions were prepared and probed by western blot with the indicated antibodies. (b) THP-1 NF-κB GFP reporter cells were either left untreated or treated with WEHI-345 (500 nM) 30 min before the addition of L18-MDP (200 ng ml−1). MFI (GFP) was measured at the indicated time points.n=3. Error bars are s.e.m. Figure 6: WEHI-345 desynchronizes NF-κB and AP-1 transcription factors. ( a ) THP-1 cells were stimulated with 200 ng ml −1 L18-MDP for the indicated time points, cytoplasmic and nuclear fractions were prepared and probed by western blot with the indicated antibodies. ( b ) THP-1 NF-κB GFP reporter cells were either left untreated or treated with WEHI-345 (500 nM) 30 min before the addition of L18-MDP (200 ng ml −1 ). MFI (GFP) was measured at the indicated time points. n =3. Error bars are s.e.m. Full size image This observation suggested that asynchronous activation of essential transcription factors by the NOD signalling pathway could result in a completely defective final response. To test this hypothesis, we used a transcription reporter that only requires activation of NF-κB. Asynchronous activation of different transcription factors should not affect transcription from such a reporter vector and as the NF-κB response is only delayed by WEHI-345 we hypothesized that transcription from this reporter vector would also only be delayed. We therefore used THP-1 cells that were stably infected with a lentiviral NF-κB GFP reporter and observed the kinetics of NF-κB activation in the presence or absence of WEHI-345. In accord with the delayed kinetics of p65 phosphorylation and translocation in the nucleus, GFP expression in cells pretreated with WEHI-345 before MDP stimulation was only delayed by 30–60 min compared with cells that were not treated with WEHI-345 and was not prevented ( Fig. 6b ). Over time, the levels of GFP increased to a similar extent in both WEHI-345-treated and untreated cells, indicating that even in the presence of WEHI-345, NF-κB is still activated following MDP stimulation. WEHI-345 blocks MDP-induced cytokine production in vivo Pharmacological inhibition of RIPK2 may be beneficial for the treatment of NOD-associated diseases such as multiple sclerosis, Blau syndrome or early-onset sarcoidosis where aberrant activation of the NOD pathway can lead to disease [10] . We therefore evaluated WEHI-345 in vivo . The pharmacokinetic properties of WEHI-345 were tested following intraperitoneal injection or oral gavage at a dose of 10 mg kg −1 ( Fig. 7a ). Absorption of both compounds was rapid and maximal plasma concentrations were detected as early as 30 min after administration and remained above the analytical limit of quantification (0.5 ng ml −1 ) for 7.5 h. Intraperitoneal injection resulted in higher maximum plasma concentrations (6.1 μM) compared to oral administration (1.2 μM). Importantly, no adverse effects after 2 daily injections over 4 days were observed. The maximal tolerated dose was determined to be 25 mg kg −1 and no pathology or changes on blood cell counts were observed at this dose. 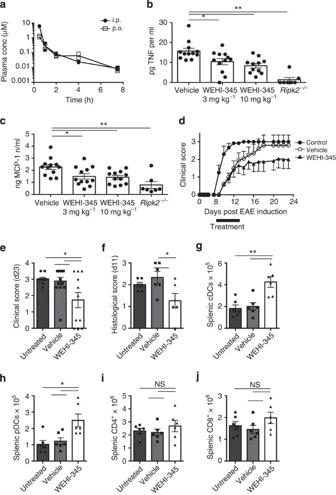Figure 7: WEHI-345 inhibits NOD signallingin vivoand has a beneficial effect on an EAE model. (a) Bioavailability of WEHI-345 after intraperitoneal (i.p.) or oral administration in non-fasted male Swiss outbred mice (n=2 for each time point). (b,c) C57BL/6 mice were pretreated for 30 min with either vehicle or WEHI-345 (100 μl, i.p. injection), followed by challenge with MDP (5 mg kg−1, i.p. injection) for 4 h. Serum levels of TNF (b) and MCP-1 (c) were determined using enzyme-linked immunosorbent assay.n=12 for all wild-type groups,n=7 forRipk2−/−. (d) EAE was induced in wild-type C57Bl/6 mice and from day 9 after disease induction, mice were treated twice daily with 20 mg kg−1WEHI-345 for 6 days. The clinical score of each mouse was assessed daily and mice were followed up to day 23. The mean clinical score ±s.e.m. of one experiment is shown. Control:n=6, vehicle:n=5, WEHI-345:n=6. (e) Clinical scores of two independent EAE experiments at d23 post disease induction. Individual scores as well as the mean score of two independent experiments are shown. Control:n=10, vehicle:n=13, WEHI-345:n=11. Control versus vehicle:P=0.620, control versus WEHI-345:P=0.017, vehicle versus WEHI-345:P=0.029. (f) Histological score of forebrain sections of untreated, vehicle- or WEHI-345-treated mice 11 days after EAE induction using an improved formulation for WEHI-345. Control:n=6, vehicle:n=6, WEHI-345:n=6. Control versus vehicle:P=0.290, control versus WEHI-345:P=0.064, vehicle versus WEHI-345:P=0.034. (g–j) splenic cellularity of untreated, vehicle or WEHI-345-treated mice at day 11 post immunization. Control:n=6, vehicle:n=6, WEHI-345:n=6. Shown are individual values, averages and error bars are s.e.m. In all panels, * indicatePvalues <0.05 and ** indicatePvalues <0.005 based on a non-paired Student’sttest. Error bars are s.e.m. Figure 7: WEHI-345 inhibits NOD signalling in vivo and has a beneficial effect on an EAE model. ( a ) Bioavailability of WEHI-345 after intraperitoneal (i.p.) or oral administration in non-fasted male Swiss outbred mice ( n =2 for each time point). ( b , c ) C57BL/6 mice were pretreated for 30 min with either vehicle or WEHI-345 (100 μl, i.p. injection), followed by challenge with MDP (5 mg kg −1 , i.p. injection) for 4 h. Serum levels of TNF (b) and MCP-1 ( c ) were determined using enzyme-linked immunosorbent assay. n =12 for all wild-type groups, n =7 for Ripk2 −/− . ( d ) EAE was induced in wild-type C57Bl/6 mice and from day 9 after disease induction, mice were treated twice daily with 20 mg kg −1 WEHI-345 for 6 days. The clinical score of each mouse was assessed daily and mice were followed up to day 23. The mean clinical score ±s.e.m. of one experiment is shown. Control: n =6, vehicle: n =5, WEHI-345: n =6. ( e ) Clinical scores of two independent EAE experiments at d23 post disease induction. Individual scores as well as the mean score of two independent experiments are shown. Control: n =10, vehicle: n =13, WEHI-345: n =11. Control versus vehicle: P =0.620, control versus WEHI-345: P =0.017, vehicle versus WEHI-345: P =0.029. ( f ) Histological score of forebrain sections of untreated, vehicle- or WEHI-345-treated mice 11 days after EAE induction using an improved formulation for WEHI-345. Control: n =6, vehicle: n =6, WEHI-345: n =6. Control versus vehicle: P =0.290, control versus WEHI-345: P =0.064, vehicle versus WEHI-345: P =0.034. ( g – j ) splenic cellularity of untreated, vehicle or WEHI-345-treated mice at day 11 post immunization. Control: n =6, vehicle: n =6, WEHI-345: n =6. Shown are individual values, averages and error bars are s.e.m. In all panels, * indicate P values <0.05 and ** indicate P values <0.005 based on a non-paired Student’s t test. Error bars are s.e.m. Full size image To test the functionality of WEHI-345 in vivo , we challenged mice with MDP after pretreatment with WEHI-345. Inflammatory markers such as TNF and MCP-1 were induced in the serum of wild-type mice 4 h after MDP challenge. Consistent with its function in vitro , administration of WEHI-345 reduced levels of TNF and MCP-1 after MDP challenge ( Fig. 7b,c ). Vehicle treatment did not have an effect compared with PBS-injected animals ( Supplementary Fig. 3a,b ). WEHI-345 ameliorates EAE in mice Recently, RIPK2 has been implicated in the pathology of chronic progressive experimental autoimmune encephalomyelitis (EAE) because Ripk2 −/− mice developed a reduced disease score compared to wild-type mice [11] . In two independent experiments, we induced EAE in wild-type C57BL/6 mice and treated with WEHI-345 twice daily (20 mg kg −1 ) for six consecutive days starting on day 9 after disease induction ( Fig. 7d , Supplementary Figure 3c , Supplementary Tables 2 and 3 ). In accord with the effect observed in Ripk2 −/− mice [11] , at the conclusion of both experiments (day 23 after disease induction), the mean disease score was significantly lower in WEHI-345-treated animals compared with untreated or vehicle-treated mice. Disease was almost completely prevented (disease score <1) in 5/11 animals treated with WEHI-345 ( Fig. 7e ). This establishes RIPK2 as a promising target for the treatment of EAE. Although there was a clear differential between WEHI-345 and vehicle-treated mice, there was nevertheless a surprising protective effect due to vehicle alone. This prompted us to test another formulation. To reduce unnecessary animal use and obtain additional insight into the role of RIPK2 kinase activity in disease progression, we combined this experiment with histological assessment of the CNS, an analysis of cellular composition of the spleen as well as analysis of inflammatory cytokines in mice at the time of onset of disease (day 11, Fig. 7f–j and Supplementary Fig. 4 ). EAE progression has been reported to be associated with the infiltration of dendritic cells (DCs) into the CNS around day 17 (ref. 11 ). We analysed the forebrain of immunized mice and detected reduced inflammatory infiltrate already at this early time point in the parenchyma in WEHI-345-treated animals ( Supplementary Fig. 4j ) and a reduced histological score in WEHI-345-treated animals ( Fig. 7f ). The increase of immune infiltrate to the brain was paralleled by a significant accumulation of splenic pDCs and cDCs in the spleen of WEHI-345-treated animals ( Fig. 7g,h ), while the amounts of CD4 + and CD8 + T cells remained unaltered ( Fig. 7i,j ), suggesting reduced recruitment of dendritic cells to the site of inflammation. We also observed a trend towards improved body weight ( Supplementary Fig. 4a ) and reduced cytokine and chemokine levels, particularly in the spleen, in WEHI-345-treated mice, indicating an overall improvement of the condition ( Supplementary Fig. 4b–i ). We have identified a novel RIPK2 kinase inhibitor, WEHI-345, which has greater specificity than previously described small-molecule kinase inhibitors, such as Erlotinib or SB-203580 that were designed to inhibit other kinases but which show some activity against RIPK2. Unbiased analysis of targets of WEHI-345 in cells and a KINOMEscan revealed that WEHI-345 has exquisite specificity for RIPK2. WEHI-345 inhibits RIPK2 activity in vitro with an IC 50 of 134 nM, while IC 50 against other RIP Kinases is greater than 10 μM. Treatment with WEHI-345 significantly inhibited IL-6 secretion from Raw 267.4 cells at 50 nM, showing a 10-fold stronger inhibition than erlotinib and gefitinib in an identical assay [22] . In cells, WEHI-345 blocked NOD-dependent cytokine production but spared necroptosis signalling mediated by RIPK1 and RIPK3. Smac-mimetic-induced activation of IL-1β, which we have recently shown involves RIPK3 and NLRP3 inflammasome activation [40] , was also unaffected by WEHI-345. Like previously described RIPK2 inhibitors, WEHI-345 targets tyrosine kinases. Although RIP kinases were originally described as serine/threonine kinases [41] , amino-acid sequence alignment suggests that RIPK2 is closely related to tyrosine kinases. We here show that WEHI-345 potently inhibits the serine/threonine kinase activity of RIPK2. One of our most striking findings with WEHI-345 was that it only caused a delay in NF-κB transcription factor activation, yet almost completely abrogated cytokine production. The p38 inhibitor SB-203580, which also inhibits RIPK2, caused a similar delay in phosphorylation events rather than a complete inhibition after NOD stimulation, supporting the idea that this phenomenon is due to RIPK2 inhibition. Notably, MDP-stimulated, NF-κB-dependent, production of GFP from a reporter vector matched the NF-κB activation profile and was only delayed reaching similar levels in WEHI-345 and control treated cells after a 45–60-min delay. This experiment shows that the NF-κB subunits that translocate into the nucleus in the presence of WEHI-345 are functional and able to induce NF-κB controlled genes. On the other hand, the timing of MDP-stimulated nuclear translocation of AP-1 transcription factors was barely affected by WEHI-345 treatment, if at all. This suggests that the delay in NF-κB signalling disrupts the tightly co-ordinated activation of the set of transcription factors that is necessary for complete transcription of inflammatory cytokines. WEHI-345 inhibited the interaction between RIPK2 and the BIR2 domain of IAPs in vitro . All mammalian IAPs: cIAP1, cIAP2 and XIAP have been shown to contribute to NOD signalling [16] , [17] , [42] and therefore WEHI-345 could inhibit NOD signalling by binding to the ATP-binding pocket of RIPK2 and altering its conformation so that RIPK2 can no longer bind to IAPs thereby preventing RIPK2 ubiquitylation and downstream signalling events. However, in cells, WEHI-345 prevented RIPK2 Ser176 autophosphorylation and because phosphorylation of kinases frequently induces a conformational change it is conceivable that phosphorylation drives a conformational change in RIPK2 that promotes IAP binding and efficient downstream signalling. Our in vitro -binding experiments were not performed in the presence of MDP and therefore support the first hypothesis. However, because we did not compare binding of the phosphorylated and unphosphorylated forms of RIPK2 to the IAPs in vitro , it is possible that phosphorylation of RIPK2 is a critical regulator of RIPK2/IAP interaction. This is another interesting area for future investigation opened up by our studies. Whether the observed delay in NF-κB activation is due to incomplete inhibition of RIPK2 kinase activity by WEHI-345 or via an alternative, RIPK2-independent pathway for NF-κB activation remains unclear. Genetic loss of RIPK2 completely abrogates phosphorylation events within the NF-κB pathway after NOD stimulation [43] ; however, unfortunately this does not address this question because ubiquitylation of RIPK2 also provides an essential platform for activation of the IKK1/IKK2/NEMO complex. Competition for the ATP-binding site of RIPK2 could result in incomplete inhibition and a delayed activation of downstream signalling. Interestingly, the use of the IAP antagonist compound A also resulted in a delay of phosphorylation events, very similar to the effect observed with WEHI-345 (ref. 44 ) and our interaction data suggest that WEHI-345 acts in a similar manner than compound A. This is further evidence that the orchestrated activation of NF-κB and other transcription factors is essential and a perturbation of these transcription factors leads to a total loss of cytokine production. Furthermore, it seems to be sufficient to block immediate signalling at the crucial 30-min time point for a complete loss of cytokine production. Finally, we provide evidence that targeting RIPK2 can be beneficial in a murine model for multiple sclerosis. WEHI-345 phenocopied the effect previously observed in RIPK2-deficient mice, even though we treated the mice only on disease onset and only for 6 days. Despite these limitations, we nevertheless prevented disease in almost half of the animals. The lack of efficacy in roughly 50% of WEHI-345-treated animals that developed disease could be due to suboptimal concentrations of WEHI-345 or that individual mice have a different stage of disease at the beginning of treatment (albeit not clinically evident yet). Surprisingly, we observed an effect on disease progression with vehicle alone, confirming the importance of such controls. To delineate the role of RIPK2, it will be necessary to find better formulations that do not have this unanticpated activity and early experiments with a different vehicle formulation suggest that this will be feasible. From a potential treatment perspective, it may, however, be interesting to follow up the role of the vehicle alone. With our second formulation, we observed a trend towards reduced cytokine production and overall health of the mice and a significant increase in the amount of dendritic cells in the spleen and decreased inflammatory infiltration in the parenchyma of the forebrain at the onset of disease. This fits with the observations of Shaw et al. [11] , who reported a dendritic cell infiltrate to the CNS that was reduced in animals deficient in the NOD signalling pathway. Our results suggest that RIPK2 inhibition results in the retention of DCs in the spleen and therefore in reduced inflammation and ameliorated disease. In summary, WEHI-345 has proven to be an excellent tool compound to specifically investigate the role of the kinase activity of RIPK2 in NOD signalling. It has revealed that asynchronous activation of transcription factors is surprisingly disruptive of cytokine production, uncovered a link between the kinase function of RIPK2 and IAP binding and finally provided evidence that targeting the RIPK2 kinase domain with a small molecule may have therapeutic utility. Synthesis of chemical compounds All non-aqueous reactions were performed in oven-dried glassware under an atmosphere of dry nitrogen, unless otherwise specified. Dry tetrahydrofuran and dichloromethane were obtained from a MBraun solvent purification system. Anhydrous acetonitrile and DMF were purchased from Sigma-Aldrich and used as supplied. All other solvents were reagent grade. Analytical thin-layer chromatography was performed on Merck silica gel 60F 254 aluminium-backed plates and were visualized by fluorescence quenching under ultraviolet light and/or a permanganate stain consisting of KMnO 4 (3.0 g), K 2 CO 3 (20 g) and 5% w/v aqueous NaOH (5 ml) in H 2 O (300 ml). Flash chromatography was performed with silica gel 60 (particle size 0.040–0.063 mm). NMR spectra were recorded on either (1) a Bruker Avance DRX 300 (FID processed on site) or (2) on a Varian INOVA 600 MHz (FID processed using ACD/NMR Processor Academic Edition) with the solvents indicated ( 1 H NMR at 300 or 600 MHz and 13 C NMR at 75 or 150 MHz). Chemical shifts are reported in p.p.m. on the δ scale and referenced to the appropriate solvent peak. Mass spectrometry was performed on a Finnigan LCQ Advantage MAX. HRMS were recorded at the Monash University Mass Spectrometry Facility using a Agilent 6220 Accurate Mass LC-TOF system with Agilent 1200 Series HPLC reference mass correction used for all accurate mass work (Ref Compd is Purine/HP0921 mix). A detailed description of the synthesis of WEHI-345 and WEHI-540 is provided in the Supplementary Material . Homology modelling of RIPK2 and in silico docking of ATP and WEHI-345 A homology model of the kinase domain of murine RIPK2 (amino acids 18–249) was constructed using MODELLER 9.11 (ref. 45 ). The threaded template was constructed using the crystal structures of human RIPK2 structure (PDB ID: 4C8B) and the murine RIPK1 structure with Necrostatin bound (PDB ID: 4ITH [28] ), resulting in a template of over 93% sequence identity. To optimize the model for docking adenosine-based compounds, ATP was manually docked into the putative nucleotide-binding site, such that it interacted via the adenosine ring to the hinge region of RIPK2 (residues Glu96 and Met98). The resultant structure was then annealed around this site for 10,000 iterations. The docking of WEHI-345 and WEHI-540 was performed using Surflex within Sybylx2.0 ( http://tripos.com/ ). A protomol was constructed around the putative ATP-binding site, with the threshold reduced to 0.28 and the bloat increased to 2 Å. Flexibility of the ligand and protein was allowed. The top 20 solutions were retained and visually analysed. Over 80% of the solutions showed a single docking cluster, thus the highest scoring of these was selected as the typical WEHI-345 docking solution. All figures were constructed in Pymol ( http://pymol.org/ ). RIPK2 biochemical assay WEHI-345 and WEHI-540 were generated in house and tested for inhibition of RIPK2 inhibition using the Transcreener ADP FP assay kit (BellBrook Labs). In brief, dose–response studies were performed in black Greiner 384-well low volume assay plates in a final volume of 20 μl. The substrate peptide (CRRKSLVGTPYWMAPE) and ATP (50 μM) were diluted in assay buffer (10 mM HEPES pH7.4, 10 mM MgCl 2 , 50 μM Na 3 VO 4 , 0.01% Tween-20, 1 mM dithiothreitol and 0.01% chicken ovalbumine) and added to the assay plates. Titrations of the test compounds were prepared in dimethylsulphoxide (DMSO) and 0.1 μl was added to the substrates by pin tool transfer (PerkinElmer). The recombinant RIPK2 enzyme (Millipore) was diluted in assay buffer and added to start the reactions, with negative controls receiving assay buffer only. After incubation for 90 min at 30 °C, the reactions were stopped by adding the detection reagent as per the manufacturer’s recommendation. Fluorescence polarization was read after 2 h on a PerkinElmer EnVision. IC 50 values were obtained by calculating per cent inhibition (%I) for each well relative to controls on the same plate and fitting the data to a four-parameter logistic equation. Conjugation of modified WEHI-345 (S4) to Sepharose beads NHS-activated Sepharose 4 Fast Flow (1 ml of packed matrix from a 50% slurry in isopropanol) was washed with DMSO (3 × 10 ml), centrifuging at 80 g for 3 min to pellet the matrix in between washes. The Sepharose was then resuspended in DMSO (1 ml) and compound S4 (20 μl of a 100 mM solution in DMSO, 2.0 μmol) was added followed by 40 μl triethylamine. The slurry was mixed by end-over-end agitation for 16 h at room temperature, protected from light. After 16 h, 70 μl ethanolamine was added to the slurry and end-over-end mixing was continued for a further 16 h at room temperature, protected from light. The slurry was then washed with DMSO (1 × 10 ml), then ethanol (3 × 10 ml). The S4 -conjugated Sepharose was then resuspended in ethanol (1 ml) to provide a 50% slurry which was transferred to a glass vial and stored at 4 °C protected from light. Liquid chromatography mass spectrometry analysis of samples of the supernatant (20 μl) taken at 1 min and 16 h indicated that >98% of compound S4 had been consumed after 16 h. Intracellular target identification THP-1 cells were cultured in lysine and arginine-free RPMI supplemented with either normal or heavy ( L -Lysine- 13 C 6 , 15 N 2 hydrochloride, L -Arginine- 13 C 6 , 15 N 4 hydrochloride) lysine and arginine (Sigma) for at least five passages before the experiment. Cells (21 × 10 6 ) of either normal or heavy labelled cells were washed in ice-cold PBS and lysed in 1.4 ml modified RIPA buffer (1% Nonident P-40, 0.1% Na deoxycholate, 150 mM NaCl, 1 mM EDTA, 50 mM Tris, pH 7.5, 5 mM NEM, phosphatase inhibitor cocktail and cOmplete Protease Inhibitor cocktail (Roche)). Lysates were separated and treated with increasing concentrations of WEHI-345 ranging from 0 to 100 μM for 20 mins at 4 °C. Following treatment, 20 μl of 50:50 S4-conjugated sepharose beads slurry were added to each lysate and mixed for 1 h at 4 °C. Following incubation, beads were spun down (4000 g , 1 min, 4 °C) and washed five times with cold lysis buffer. Light and heavy samples were then combined and the beads were diluted in 8 M and 100 mM Tris-HCl followed by protein digestion with 2 μg trypsin according to the previously published FASP protocol [46] . After 16 h of digestion, peptides were eluted from the filters with 50 mM ammonium bicarbonate buffer. Peptides were acidified using 1% formic acid and purified on C18 StageTips (Thermo Scientific) and subjected to LC-MS/MS for relative protein abundancies (see below). LC-MS/MS and data analysis Peptides were separated by reverse-phase chromatography on a Waters 500 mm column (ID 75 μm, 1.8 μm Acquity HSS T3), using a nano-flow HPLC (M-class, Waters). The HPLC was coupled to an Impact II UHR-QqTOF mass spectrometer (Bruker) using a CaptiveSpray source and nanoBooster at 0.20 Bar using acetonitrile. Peptides were loaded directly onto the column with buffer A (3% acetonitrile, 0.1% formic acid) and eluted with a 120 min linear gradient from 3 to 35% buffer B (99.9% acetonitrile, 0.1% formic acid). Mass spectra were acquired in a data-dependent manner, with an automatic switch between MS and MS/MS scans using a 2.5-s duty cycle and 2 Hz MS1 spectra rate followed by MS/MS scans at 4–16 Hz dependent on precursor intensity for the remainder of the cycle. MS spectra were acquired between a mass range of 150–2,200 m/z . Peptide fragmentation was performed using CID. MS files were analysed by MaxQuant version 1.5.0.25. MS spectra were searched by the Andromeda search engine against protein sequences obtained from the Uniprot, Swissprot and Ensembl knowledge bases. The maximum number of isotopic labelled amino acids was set at three. MaxQuant analysis included an initial search with a precursor mass tolerance of 0.07 Da. In the main search, precursor mass tolerance was 0.006 Da and fragment mass tolerance was 40 ppm. The search included variable modifications of oxidation (methionine), amino-terminal acetylation, carbamidomethyl (cysteine), N -ethylmaleimide (cysteine), GlyGly (lysine) and phosphorylation (serine, threonine and tyrosine). Minimum peptide length was set to seven amino acids and a maximum of two missed cleavage sites with strict trypsin specificity. The false discovery rate was set to 0.01 for PSM and protein identifications. KINOMEscan KINOMEscans were performed by LeadHunter discovery services. In brief, streptavidin-coated magnetic beads were mixed with biotinylated small-molecule ligands to generate affinity resins for the assay. After blocking, binding reactions were assembled by combining DNA tagged kinases, inhibitors and liganded affinity beads. The assay plates were incubated at room temperature for 1 h with constant shaking and the affinity beads were washed. The beads were then resuspended in elution buffer and incubated at room temperature for 30 min with shaking. The kinase concentration in the eluates was measured by a quantitative, precise and ultrasensitive quantitative PCR (qPCR). The per cent inhibition was calculated by measuring the amount of kinase captured on the solid support as a function of the test compound concentration. Cell culture and stimulation HeLa, Raw 264.7 and MDFs were maintained in DMEM supplemented with 10% fetal calf serum (FCS) and antibiotics. THP-1 cells were maintained in RPMI medium supplemented with 10% FCS and antibiotics. BMDMs were generated from wild-type and Ripk2 −/− mice. In brief, the bone marrow from tibiae and femura were cultured for 6 days in DMEM (Invitrogen) supplemented with 10% FCS (GIBCO) and 20% L929 supernatant and antibiotics (Penicillin, Streptomycin, GIBCO) [47] . After 6 days, the cells were detached using Trypsin and replated in 24-,12- or six-well plates. On the day of stimulation, the cells were either primed with murine interferon-γ (5 ng ml −1 , R&D Systems) for 2 h before the addition of MDP (10 μg ml −1 , Bachem) or directly stimulated with L18-MDP (200 ng ml −1 , Invivogen). Fc-hTNF (100 nM), Compound A (500 nM, TetraLogic Pharmaceuticals) or ultrapure LPS (25 ng ml −1 , Invivogen) was added to unprimed BMDMs. For inflammasome stimulation, BMDMs were primed with ultrapure LPS (20 ng ml −1 ) for 3 h followed by stimulation with Alum (300 μg ml −1 , 5.5 h, Thermo Scientific), ATP (5 mM, 1.5 h, Sigma), Compound A (500 nM, 5.5 h) or Staurosporine (1 μM, 5.5 h, Sigma). Necroptosis was induced by treatment with a mix of hFcTNF (100 ng ml −1 ), Compound A (500 nM) and Q-VD-Oph (10 μM, MP Biochemicals). Necrostatin-1 (50 μM, Sigma) was added 30 min before necroptosis induction. All cells were cultured in 10% CO 2 at 37 °C in a humified incubator [47] . FACS analysis For cell death assays, MDFs were stained with propidium iodide and fluorescence was assessed on a FACS Calibur (BD). Splenic cell populations were determined by mechanical disruption of one third of the spleen and staining of the cells with anti-CD4 (RM4–5, BD Bioscience), anti-CD8 (53-6.7, BD Bioscience) anti-SiglecH (ebio440c, eBioscience) and anti-CD11c (HL3, BD Bioscience). All antibodies were used at a dilution of 1:200. cDCs were defined as CD11c high , SiglecH + , pDCs were defined as CD11c intermediate , SiglecH + . Monocyte isolation and culture Heparinized blood of CCR2-CFP reporter mice [48] was suspended in red blood cell lysis buffer, centrifuged and the cell pellet was washed and resuspended in PBS containing 2% FCS. Washed cells were then stained for cell surface markers CD11b, Ly6C and Ly6G. CCR2 expression was used for separation of Ly6C + CCR2 + and Ly6C − CCR2 − monocytes by FACS: for monocyte culture, 2 × 10 4 cells were cultured in 0.2 ml 10% FCS RPMI (Invitrogen) in a 96-well round bottom plate in the absence or presence of 5 × 10 6 Listeria monocytogenes for 24 h. Culture supernatants were assayed for cytokines and chemokines as described above. Purification of ubiquitin conjugates GST-Tandem Ubiquitin Binding Entities (TUBE1, Lifesensors) were used to purify ubiquitin conjugates from THP-1 cells according to the manufacturer’s recommendations [49] . THP-1 were lysed in ice-cold lysis buffer (100 μl per 10 6 cells) and lysates were incubated with TUBEs and affinity resin for 2 h on ice on a rotating wheel at 4 °C before 3 × washing in cold PBS-Tween. Washed beads were resuspended in 1 × SDS sample buffer and subjected to western blotting. Western blotting After stimulation, cells were directly lysed in 1 × SDS sample buffer. DNA was degraded with repeated freeze/boil cycles. Nuclear and cytoplasmic fractionation was performed using NE-PER nuclear protein extraction kit (Pierce) according to the manufacturer’s instructions. Total lysates or cytoplasmic and nuclear fractions were run on SDS/polyacrylamide gel electrophoresis gradient gels, transferred to polyvinylidene fluoride or nitrocellulose membrane and blotted with antibodies against total Phospho-p65, ERK, phospho-ERK, phospho- IκBα, total IκBα, phospho-JNK1/2, total JNK1/2, cJun, cFos, GAPDH (all Cell Signalling), Ubiquitin (Imgenex), RIPK2, total p65, JunB, p50, RelB, Lamin A/C (Santa Cruz) and β-actin (Sigma). All antibodies were used at a dilution of 1:1,000 except anti-phospho IκBα (1:2,000), anti-RIPK2, anti-JunB, anti-p50 (all 1:500) and anti-β-actin (1:5,000). Images have been cropped for presentation. Full-size images are presented in Supplementary Figs 5–7 . NF-κB activity assay THP-1 cells were stably transfected with an NF-κB GFP reporter (pTRH NF-κB, System Biosciences). Cells were left untreated or stimulated with either WEHI-345 or WEHI-450, followed by stimulation with L18-MDP or C12-iE-DAP (Invivogen) for different time points. NF-κB activity was assessed by the mean fluorescence intensity of green cells using Weasel software (WEHI). Cytokine measurement by ELISA Cytokines from cell culture supernatants or mouse serum were either measured using Ready-SET-Go! ELISA kits from eBioscience or by Multiplex analysis (BioRad) according to the manufacturer’s instructions. Mouse sera were diluted up to 1:10 and cell culture supernatants up to 1:2 for TNF and IL-6 and 1:20 for MCP-1 measurements. qPCR Total RNA from cultured BMDMs or THP-1 cells at indicated time points was isolated using TRIZOL or the RNeasy Mini Kit (Quiagen) according to the manufacturer’s instructions. Complementary DNA was synthesized using SuperScript III reverse Transcriptase (Invitrogen) and oligo(d)t primers, in the presence or RNasin (Promega). qPCR was performed using Brilliant III Ultra-Fast SYBR Green qPCR Master Agilent Technologies). Primer sequences were Sense mmTnf 5′-CATCTTCTCAAAATTCGAGTGACAA-3′; Anti-Sense mmTnf 5′-TGGGAGTAGA-CAAGGTACAACCC-3′; Sense mmIl6 5′-CTGCAAGAGACTTCCATCCAGTT-3′; Anti-Sense mmIl6 5′-GAAGTAGGGAAGGCCGTGG-3′; Sense hsIL8 5′-GTTCCACTGTGCCTTGGTTT-3′; Anti-Sense hsIL8 5′-GCTTCCACATGTCCTCACAA-3′; Sense hsTNF 5′-TGCTGCAGGACTTGAGAAGA-3′; Anti-Sense hsTNF 5′-GAGGAAGGCCTAAGGTCCAC-3′; Sense hsA20 5′-ATGCACCGATACACACTGGA-3′; Anti-Sense hsA20 5′-GGATGATCTCCCGAAACTGA-3′; Sense hsIL-1 β 5′-AAGCTGATGGCCCTAAACAG-3′; Anti-Sense hsIL-1 β 5′-AGGTGCATCGTGCACATAAG-3′; Hypoxanthine phosphoribosyltransferase ( HPRT ; used as reference for normalization) hsHPRT sense 5′-AGCCAGACTTTGTTGGATTTG-3′ hsHPRT anti-sense 5′-TTTACTGGCGATGTCAATAGG-3′. RIPK2-IAP interaction studies pGEX-6 P-3 XIAP BIR2, pGEX-6 P-3 cIAP1 BIR2 or pGEX-6 P-1 were transformed into BL21 (DE3+) bacteria and grown in Super broth overnight at 37 °C. Overnight culture was diluted 1:10 and grown until OD 595 was 0.8. Isopropylthiogalactoside (0.3 mM, Sigma) was added for 4 h at 30 °C. Cells were pelleted and resuspended in Buffer A (50 mM Tris pH 8.0, 50 mM NaCl, 1 mM EDTA, 1 mM DTT, 10% glycerol) and sonicated. After centrifugation at 21,000 g for 30 min, the supernatant was incubated with glutathione sepharose 4B (GE Healthcare) for 4 h, washed five times with Buffer A, and eluted 2 × 45 min with 10 mM reduced glutathione in Buffer A at 4 °C. Elutions were dialysed into Buffer A for storage at −80 °C. For pull-down experiments, THP-1 cells (10–20 million cells per sample) were washed in PBS and lysed in 0.5 ml MELB (20 mM Hepes pH 7.5, 50 mM KCl, 2.5 mM MgCl 2 , 1 mM EDTA, 250 mM sucrose, 0.025% digitonin) with protease inhibitors. After spinning at 13,000 r.p.m. for 5 min, lysates were added directly to 50 μl packed glutathione sepharose beads prebound with 60 μg GST-BIR2 of human cIAP1, GST-BIR2 of human XIAP, or GST alone. In competition assays, WEHI-345 was added to cells in culture (2 μM) for 30 min at 37 °C before lysis. After incubating on a rotating wheel at 4 °C (4 h for competition studies, overnight for compound elution studies), beads were washed 3 × with 0.5 ml MELB without sucrose or digitonin. Beads were either eluted with 2 × 0.75 μl 25 mM glycine pH 2.5 or with 50 μM WEHI-345 or compound A. Pharmacokinetics Pharmacokinetics of WEHI-345 and WEHI-540 were assessed in non-fasted male Swiss outbred mice after intraperitoneal injection or oral gavage (both 100 μl). Triplicate aliquots were taken from the middle of each bulk formulation before dosing to confirm concentration. Blood samples were taken at 0.5, 1, 2, 4 and 7.5 h by submandibular bleed or heart puncture. A maximum of two blood samples per mouse were taken. Drug concentrations in the serum were determined by LC-MS. Mouse experiments All mouse experiments were performed according to the guidelines of the animal ethics committee of WEHI, ethics approval 2011.014 and 2014.004. Sex- and age-matched C57Bl/6 mice, were used for all in vivo experiments. Bone marrow was harvested from wild-type or Ripk2 −/− mice of various ages and both sexes. Ripk2 −/− mice were a kind gift of Professor R. Flavell and were generated using 129S1/Sv-derived embryonic stem cells and have been backcrossed to C57Bl/6 mice for at least 10 generations. All mice were kept in microisolator cages (up to six mice per cage) and had access to food and water ad libitum . In vivo MDP challenge Six–10-week-old C57Bl/6 female mice were injected intraperitoneally with WEHI-345 or vehicle control (40% polyethyleneglycol 400 (Sigma), 20% Koliphor HS15 (Sigma), 0.83% benzylalcohol (Sigma)) in a 100 μl inoculum. After 30 min, mice were challenged with 100 μg MDP (Bachem) or with PBS control by another intraperitoneal injection (100 μl). The mice were killed by CO 2 asphyxiation 4 h after MDP treatment and the blood was harvested by heart puncture. Induction and treatment of EAE For the induction of EAE, 8-week-old C57BL/6 male mice were injected subcutaneously with 100 μg MOG 35–55 peptide (Mimotopes) emulsified in complete Freund’s adjuvant supplemented with 5 mg ml −1 heat-killed Mycobacterium tuberculosis H37RA (Difco). Mice also received 300 ng pertussis toxin (Sigma) intravenously on days 0 and 2 (ref. 50 ). For disease score studies, mice were either left untreated or intraperitoneally injected twice daily with vehicle or 20 mg kg −1 WEHI-345, for six consecutive days from day 9 after immunization. Neurological impairment was scored daily: 0, no clinical signs; 1, limp tail; 2, hind limb weakness; 3, hind limb paralysis; 3.5, euthanized mouse due to disease score >3 (according to the guidelines of the AEC of WEHI). For the short time study, the vehicle was changed to 12% Capisol pH 4.0 and treatment was started at day 8 post immunization. Two daily doses of 20 mg kg −1 WEHI-345 or vehicle was administered and mice were euthanized 2 h after the last treatment on day 11 post immunization. Histological analysis of EAE Eleven days post immunization, the brains of untreated, vehicle-treated or WEHI-345-treated mice were fixed in 4% paraformaldehyde for at least 48 h. Three haematoxylin and eosin-stained sections of each brain, each 30–50 μm apart, were analysed by a double-blinded individual and a histological score for each slide was determined based on cellular infiltration to the parenchyma of the forebrain. The histological score per mouse is the average of the three sections of one mouse. Histological scores: 0, minimal to no cellular infiltrate in parenchyma; 1, mild cellular infiltrate in parenchyma; 2, moderate cellular infiltrate to parenchyma; 3, severe cellular infiltrate in parenchyma. Statistical analysis Unless stated otherwise, non-paired Student’s t -tests were performed for statistical analysis. P values <0.05 are indicated by * P values <0.005 by ** P values <0.1 were considered as a trend. How to cite this article: Nachbur, U. et al. A RIPK2 inhibitor delays NOD signalling events, yet prevents inflammatory cytokine production. Nat. Commun. 6:6442 doi: 10.1038/ncomms7442 (2015).